Identification and molecular characterization of a new ovarian cancer susceptibility locus at 17q21.31 Epithelial ovarian cancer (EOC) has a heritable component that remains to be fully characterized. Most identified common susceptibility variants lie in non-protein-coding sequences. We hypothesized that variants in the 3′ untranslated region at putative microRNA (miRNA)-binding sites represent functional targets that influence EOC susceptibility. Here, we evaluate the association between 767 miRNA-related single-nucleotide polymorphisms (miRSNPs) and EOC risk in 18,174 EOC cases and 26,134 controls from 43 studies genotyped through the Collaborative Oncological Gene–environment Study. We identify several miRSNPs associated with invasive serous EOC risk (odds ratio=1.12, P =10 −8 ) mapping to an inversion polymorphism at 17q21.31. Additional genotyping of non-miRSNPs at 17q21.31 reveals stronger signals outside the inversion ( P =10 −10 ). Variation at 17q21.31 is associated with neurological diseases, and our collaboration is the first to report an association with EOC susceptibility. An integrated molecular analysis in this region provides evidence for ARHGAP27 and PLEKHM1 as candidate EOC susceptibility genes. Genome-wide association studies (GWAS) have identified hundreds of genetic variants conferring low penetrance susceptibility to cancer [1] . More than 90% of these variants lie in non protein-encoding sequences including non-coding RNAs and regions containing regulatory elements (that is, enhancers, promoters, untranslated regions (UTRs)) [1] . The emerging hypothesis is that common variants within non-coding regulatory regions influence expression of target genes, thereby conferring disease susceptibility [1] . MicroRNAs (miRNAs) are short non-coding RNAs that regulate gene expression post-transcriptionally by binding primarily to the 3′UTR of target messenger RNA (mRNA), causing translational inhibition and/or mRNA degradation [2] , [3] , [4] . MiRNAs have been shown to have a key role in the development of epithelial ovarian cancer (EOC) [2] . We [5] , [6] and others [7] have found evidence that various miRNA-related single-nucleotide polymorphisms (miRSNPs) are associated with EOC risk, suggesting they may be key disruptors of gene function and contributors to disease susceptibility [8] , [9] . However, studies of miRSNPs that affect miRNA–mRNA binding have been restricted by small sample sizes, and therefore have limited statistical power to identify associations at genome-wide levels of significance [7] , [8] , [9] . Large-scale studies and more systematic approaches are warranted to fully evaluate the role of miRSNPs and their contribution to disease susceptibility. Here, we use the in silico algorithms, TargetScan [10] , [11] and Pictar [12] , [13] to predict miRNA:mRNA-binding regions involving genes and miRNAs relevant to EOC, and align identified regions with SNPs in the Single Nucleotide Polymorphism database (dbSNP) (Methods). We then genotype 1,003 miRSNPs (or tagging SNPs with r 2 >0.80) in 18,174 EOC cases and 26,134 controls from 43 studies from the Ovarian Cancer Association Consortium (OCAC) ( Supplementary Table S1 ). Genotyping was performed on a custom Illumina Infinium iSelect array designed as part of the Collaborative Oncological Gene–environment Study (COGS), an international effort that evaluated 211,155 SNPs and their association with ovarian, breast and prostate cancer risk. Our investigation uncovers 17q21.31 as a new susceptibility locus for EOC, and we provide insights into candidate genes and possible functional mechanisms underlying disease development at this locus. Association analyses Seven hundred and sixty-seven of the 1,003 miRSNPs passed genotype quality control (QC) and were evaluated for association with invasive EOC risk; most of the miRSNPs that failed QC were monomorphic (see Methods). Primary analysis of 14,533 invasive EOC cases and 23,491 controls of European ancestry revealed four strongly correlated SNPs ( r 2 =0.99; rs1052587, rs17574361, rs4640231 and rs916793) that mapped to 17q21.31 and were associated with increased risk (per allele odds ratio (OR)=1.10, 95% confidence interval (CI) 1.06–1.13) at a genome-wide level of significance (10 −7 ); no other miRSNPs had associations stronger than P <10 −4 ( Supplementary Fig. S1 ). 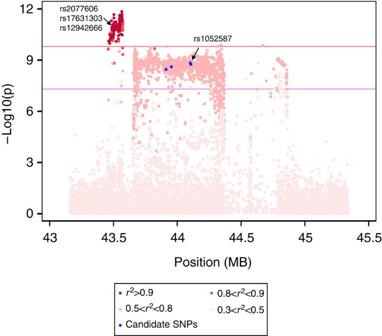Figure 1: Regional association plot for genotyped and imputed SNPs at 17q21.31. The middle portion of the plot contains the region of the inversion polymorphism (ch 17: 43,624,578–44,525,051, hg build 37), with the four blue dots representing the candidate miRSNPs (rs4640231, rs1052587 and rs17574361) and the tagSNP, rs916793. rs1052587 in the 3′UTR ofMAPThas the strongest signal (P=4.6 × 10−8) among the miRSNPs. The cluster on the left side of the plot (around 43.5 MB) contains highly correlated SNPs (r2=0.99), including three directly genotyped intronic SNPs, rs2077606 and rs17631303 inPLEKHM1(P=3.9 × 10−10andP=4.7 × 10−10, respectively), and rs12942666 inARHGAP27(P=1.0 × 10−9). The LD between each plotted SNP and the top-ranked SNP in the region with the best clustering, rs12942666, is depicted by the colour scheme; the deeper the colour red, the stronger the correlation between the plotted SNP and rs12942666. The top miRSNP, rs1052587, is moderately correlated (r2=0.76) with rs2077606, rs17631303 and rs12942666 in our study population (n=8,371 invasive serous cases andn=23,491 controls, of European ancestry). The most significant association was for rs1052587 ( P =1.9 × 10 −7 ), and effects varied by histological subtype, with the strongest effect observed for invasive serous EOC cases (OR=1.12, P =4.6 × 10 −8 ) ( Table 1 ). No heterogeneity in ORs was observed across study sites ( Supplementary Fig. S2 ). Table 1 Tests of association by histological subtype for directly genotyped and imputed SNPs at 17q21.31 most strongly associated with invasive epithelial ovarian cancer risk among Europeans. Full size table Rs1052587, rs17574361 and rs4640231 reside in the 3′UTR of microtubule-associated protein tau ( MAPT) , KAT8 regulatory NSL complex subunit 1 ( KANSL1/KIAA1267) and corticotrophin-releasing hormone receptor 1 ( CRHR1) genes, at putative binding sites for miR-34a, miR-130a and miR-34c, respectively. The fourth SNP, rs916793, is perfectly correlated with rs4640231 and lies in a non-coding RNA, MAPT -antisense 1. 17q21.31 contains a ~900-kb inversion polymorphism [14] (ch 17: 43,624,578–44,525,051 MB, human genome build 37), and all three miRSNPs and the tagSNP are located within the inversion ( Fig. 1 ). Figure 1: Regional association plot for genotyped and imputed SNPs at 17q21.31. The middle portion of the plot contains the region of the inversion polymorphism (ch 17: 43,624,578–44,525,051, hg build 37), with the four blue dots representing the candidate miRSNPs (rs4640231, rs1052587 and rs17574361) and the tagSNP, rs916793. rs1052587 in the 3′UTR of MAPT has the strongest signal ( P =4.6 × 10 −8 ) among the miRSNPs. The cluster on the left side of the plot (around 43.5 MB) contains highly correlated SNPs ( r 2 =0.99), including three directly genotyped intronic SNPs, rs2077606 and rs17631303 in PLEKHM1 ( P =3.9 × 10 −10 and P =4.7 × 10 −10 , respectively), and rs12942666 in ARHGAP27 ( P =1.0 × 10 −9 ). The LD between each plotted SNP and the top-ranked SNP in the region with the best clustering, rs12942666, is depicted by the colour scheme; the deeper the colour red, the stronger the correlation between the plotted SNP and rs12942666. The top miRSNP, rs1052587, is moderately correlated ( r 2 =0.76) with rs2077606, rs17631303 and rs12942666 in our study population ( n =8,371 invasive serous cases and n =23,491 controls, of European ancestry). Full size image Chromosomes with the non-inverted or inverted segments of 17q21.31, respectively, known as haplotype 1 (H1) and haplotype 2 (H2), represent two distinct lineages that diverged ~3 million years ago and have not undergone any recombination event [14] . The four susceptibility alleles identified here reside on the H2 haplotype that is reported to be rare in Africans and East Asians, but is common (frequency >20%) and exhibits strong linkage disequilibrium (LD) among Europeans [14] , consistent with our findings. The H2 haplotype has a frequency of 22% among European women in our primary analysis ( Table 1 ) but only 3.2 and 0.3% among Africans (151 invasive cases, 200 controls) and Asians (716 invasive cases, 1573 controls), respectively. To increase genomic coverage at this locus, we evaluated an additional 142 non-miRSNPs at 17q21.31 that were also genotyped as a part of COGS in the same series of OCAC cases and controls. We also imputed genotypes using data from the 1000 Genomes Project [15] . These approaches identified a second cluster of strongly correlated SNPs ( r 2 >0.90) in a distinct region proximal to the inversion (centred at chromosome 17: 43.5 MB, human genome build 37) that was more significantly associated with the risk of all invasive EOCs ( P =10 −9 ) and invasive serous EOC specifically ( P =10 −10 ) than the cluster of identified miRSNPs ( Fig. 1 ). Association results and annotation for SNPs in this second cluster are shown in Supplementary Table S2 ; this cluster includes three directly genotyped SNPs (rs2077606, rs17631303 and rs12942666), with the strongest association observed for rs2077606 among all invasive cases (OR=1.12, 95% CI: 1.08–1.16, P =7.8 × 10 −9 ) and invasive serous cases (OR=1.15, 95% CI: 1.12–1.19, P =3.9 × 10 −10 ). These SNPs were chosen for genotyping in COGS because they had shown evidence of association as modifiers of EOC risk in BRCA1 gene mutation carriers by the Consortium of Investigators of Modifiers of BRCA1/2 (CIMBA) [16] . Several imputed SNPs in strong LD ( r 2 >0.90) were more strongly associated with risk than their highly correlated genotyped SNPs ( Supplementary Table S2 ). This risk-associated region at 17q21.31 is distinct from a previously reported ovarian cancer susceptibility locus at 17q21 (ref. 17 ); neither the genotyped nor the imputed SNPs we report here are strongly correlated (maximum r 2 =0.01) with SNPs from the 17q21 locus (spanning 46.2–46.5 MB, build 37). Genotype clustering was poor for rs2077606, but clustering was good for its correlated SNP, rs12942666 ( r 2 =0.99) and so results for this SNP are presented instead ( Supplementary Fig. S3 ; Table 1 ). Subgroup analysis revealed marginal evidence of association for rs12942666 with endometrioid ( P =0.04), but not mucinous or clear cell EOC subtypes ( Table 1 ), and results were consistent across studies ( Supplementary Fig. S4 ). Rs12942666 is correlated with the top-ranked miRSNP, rs1052587 ( r 2 =0.76) ( Fig. 1 ). To evaluate whether associations observed for rs12942666 and rs1052587 represented independent signals, stepwise logistic regression was used; only rs12942666 was retained in the model. This suggests that the cluster which includes rs12942666 is driving the association with EOC risk that was initially identified through the candidate miRSNPs. Functional and molecular analyses To evaluate functional evidence for candidate genes, risk-associated SNPs, and regulatory regions at 17q21.31, we examined a 1-MB region centred on rs12942666 using a combination of locus-specific and genome-wide assays and in silico analyses of publicly available data sets, including The Cancer Genome Atlas (TCGA) Project [18] (see Methods). Rs12942666 and many of its correlated SNPs lie within introns of Rho GTPase activating protein 27 ( ARHGAP27 ) or its neighbouring gene, pleckstrin homology domain containing family M (with RUN domain) member 1 ( PLEKHM1 ) ( Supplementary Table S2 ). There are another 15 known protein-coding genes within the region: KIF18B, C1QL1, DCAKD, NMT1, PLCD3, ABCB4, HEXIM1, HEXIM2, FMNL1, C17orf46, MAP3K14, C17orf69, CRHR1, IMP5 and MAPT ( Fig. 2a ). 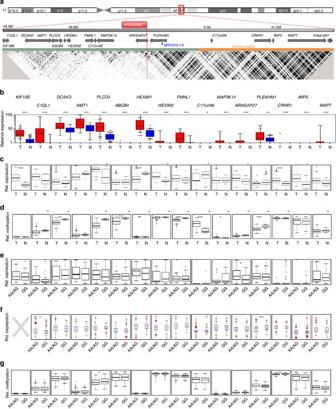Figure 2: Expression and methylation analyses at the 17q21.31 ovarian cancer susceptibility locus. (a) Genomic map and LD structure. The location and approximate size of 17 known protein-coding genes (grey) and one microRNA (blue) in the region are shown relative to the location of rs12942666. Orange indicates the location of the inversion polymorphism, and green indicates the region outside the inversion. (b) Gene expression (EOC and normal cell lines). Gene expression analysis in epithelial ovarian cancer (EOC) cell lines (T;n=51) compared with normal ovarian surface epithelial cells (OSECs) and fallopian tube secretory epithelial cells (FTSECs) (N;n=73) (*P<0.05, **P<0.01, ***P<0.001). (c) Gene expression (primary EOCs and normal tissue). Boxplots of The Cancer Genome Atlas (TCGA) Affymetrix U133A-array-based gene expression in primary high-grade serous ovarian tumours (T;n=568) and normal fallopian tube tissues (N;n=8). Where data were not available in TCGA, gene expression data from the Gene Expression Omnibus series GSE18520 data set containing 53 high-grade serous tumours and 10 normal ovarian tissues are shown (indicated by a red asterisk). (d) Methylation (primary tumours and normal tissue). Methylation analysis of 106 high-grade serous ovarian tumours compared with normal ovarian tissues (n=7). Methylation data were generated for CpG site(s) associated with each gene using the Illumina 450 methylation array. Pairwise analysis of methylation for an individual CpG for each gene is based on the CpG with most significant inverse relationship to gene expression (that is,cisnegative), for a subset of 43 tumours having available gene expression data. Statistically significantcis-negative probes are indicated by a red open circle. (e) eQTL analysis (OSECs/FTSECs). eQTL analysis comparing expression of each gene to genotype for the most statistically significant SNP at 17q21.31 (rs12942666), for 73 normal OSEC/FTSEC lines. Data are presented as box plots comparing expression levels in cases carrying rare homozygotes/heterozygotes, with cases homozygous for the common allele. (f) eQTL analysis (primary EOCs). eQTL analysis comparing expression of each gene by genotype using level 3 gene expression profiling data from Agilent 244K custom arrays and level 2 genotype data from the Illumina 1M-Duo BeadChip for 568 high-grade serous ovarian cancer patients from TCGA. In all panels *P<0.05, **P<0.01, ***P<0.001. Grey X’s indicate data not available. Here, genotype data for rs2077606 is used (rather than rs12942666) because rs12942666 was not genotyped in the TCGA data set. (g) Methylation quantitative trait locus (mQTL) analysis (primary EOCs). mQTL analysis showing methylation status in 227 high-grade serous EOCs relative to rs12942666 genotype. Figure 2: Expression and methylation analyses at the 17q21.31 ovarian cancer susceptibility locus. ( a ) Genomic map and LD structure. The location and approximate size of 17 known protein-coding genes (grey) and one microRNA (blue) in the region are shown relative to the location of rs12942666. Orange indicates the location of the inversion polymorphism, and green indicates the region outside the inversion. ( b ) Gene expression (EOC and normal cell lines). Gene expression analysis in epithelial ovarian cancer (EOC) cell lines (T; n =51) compared with normal ovarian surface epithelial cells (OSECs) and fallopian tube secretory epithelial cells (FTSECs) (N; n =73) (* P <0.05, ** P <0.01, *** P <0.001). ( c ) Gene expression (primary EOCs and normal tissue). Boxplots of The Cancer Genome Atlas (TCGA) Affymetrix U133A-array-based gene expression in primary high-grade serous ovarian tumours (T; n =568) and normal fallopian tube tissues (N; n =8). Where data were not available in TCGA, gene expression data from the Gene Expression Omnibus series GSE18520 data set containing 53 high-grade serous tumours and 10 normal ovarian tissues are shown (indicated by a red asterisk). ( d ) Methylation (primary tumours and normal tissue). Methylation analysis of 106 high-grade serous ovarian tumours compared with normal ovarian tissues ( n =7). Methylation data were generated for CpG site(s) associated with each gene using the Illumina 450 methylation array. Pairwise analysis of methylation for an individual CpG for each gene is based on the CpG with most significant inverse relationship to gene expression (that is, cis negative), for a subset of 43 tumours having available gene expression data. Statistically significant cis -negative probes are indicated by a red open circle. ( e ) eQTL analysis (OSECs/FTSECs). eQTL analysis comparing expression of each gene to genotype for the most statistically significant SNP at 17q21.31 (rs12942666), for 73 normal OSEC/FTSEC lines. Data are presented as box plots comparing expression levels in cases carrying rare homozygotes/heterozygotes, with cases homozygous for the common allele. ( f ) eQTL analysis (primary EOCs). eQTL analysis comparing expression of each gene by genotype using level 3 gene expression profiling data from Agilent 244K custom arrays and level 2 genotype data from the Illumina 1M-Duo BeadChip for 568 high-grade serous ovarian cancer patients from TCGA. In all panels * P <0.05, ** P <0.01, *** P <0.001. Grey X’s indicate data not available. Here, genotype data for rs2077606 is used (rather than rs12942666) because rs12942666 was not genotyped in the TCGA data set. ( g ) Methylation quantitative trait locus (mQTL) analysis (primary EOCs). mQTL analysis showing methylation status in 227 high-grade serous EOCs relative to rs12942666 genotype. Full size image To evaluate the likelihood that one or more genes within this region represent target susceptibility gene(s), we first analysed expression, copy number variation and methylation involving these genes in EOC tissues and cell lines ( Fig. 2b–g ; Supplementary Tables S3 and S4 ). Most genes showed significantly higher expression ( P <10 −4 ) in EOC cell lines versus normal ovarian cancer precursor tissues (OCPTs); ARHGAP27 showed the most pronounced difference in gene expression between cancer and normal cells ( P =10 −16 ) ( Fig. 2b and Supplementary Table S3 ). For nine genes, we also found overexpression in primary high-grade serous (HGS) EOC tumours versus normal ovarian tissue in at least one of two publicly available data sets, TCGA series of 568 tumours [18] and/or the Gene Expression Omnibus series GSE18520 data set consisting of 53 tumors [19] ( Fig. 2c and Supplementary Table S3 ). Analysis of DNA copy number variation in TCGA revealed frequent loss of heterozygosity in this region rather than copy number gains ( Supplementary Fig. 5a–b ; Supplementary Methods ). We observed significant hypomethylation ( P <0.01) in ovarian tumours compared to normal tissues for DCAKD, PLCD3, ACBD4 , FMNL1 and PLEKHM1 ( Fig. 2d and Supplementary Table S4 ), which is consistent with the overexpression observed for DCAKD , PLCD3 and FMNL1 . Taken together, these data suggest that the mechanism underlying overexpression may be epigenetic rather than based on copy number alterations. We evaluated associations between genotypes for the top risk SNP rs12942666 (or a tagSNP) and expression of all genes in the region (expression quantitative trait locus (eQTL) analysis) in normal OCPTs, lymphoblastoid cell lines and primary ovarian tumours from TCGA. The only significant eQTL association observed ( P <0.05) in normal OCPTs was for ARHGAP27 ( P =0.04) ( Fig. 2e ; Supplementary Table S3 ). Because rs12942666 was not genotyped in tissues analysed in TCGA, we used data for its correlated SNP rs2077606 ( r 2 =0.99) to evaluate eQTLs in tumour tissues. Rs2077606 genotypes were strongly associated with PLEKHM1 expression in primary HGS-EOCs ( P =1 × 10 −4 ) ( Fig. 2f ; Supplementary Table S3 ). We also detected associations between rs12942666 (and rs2077606) genotypes and methylation for PLEKHM1 and CRHR1 in primary ovarian tumours ( P =0.020 and 0.001, respectively) using methylation quantitative trait locus analyses ( Fig. 2g ; Supplementary Table S4 ). Finally, the Catalogue of Somatic Mutations in Cancer database [20] showed that nine genes in the region, including PLEKHM1 , have functionally significant mutations in cancer, although for most genes mutations were not reported in ovarian carcinomas ( Supplementary Table S3 ). Taken together, these data suggest that several genes at the 17q21.31 locus may have a role in EOC development. The risk-associated SNPs we identified fall within non-coding DNA, suggesting the functional SNP(s) may be located within an enhancer, insulator or other regulatory element that regulates expression of one of the candidate genes we evaluated. One hypothesis emerging from these molecular analyses is that rs12942666 (or a correlated SNP) mediates regulation of PLEKHM1 , a gene implicated in osteopetrosis and endocytosis [21] and/or ARHGAP27 , a gene that may promote carcinogenesis through dysregulation of Rho/Rac/Cdc42-like GTPases [22] . To identify the most likely candidate for being the causal variant at 17q21.31, we compared the difference between log-likelihoods generated from un-nested logistic regression models for rs12942666 and each of 198 SNPs in a 1-MB region featured in Supplementary Table 2 . As expected, the log-likelihoods were very similar due to the strong LD; no SNPs emerged as having a likelihood ratio >20 for being the causal variant. To explore the possible functional significance of rs12942666 and strongly correlated variants ( r 2 >0.80), we then generated a map of regulatory elements around rs12942666 using ENCyclopedia of DNA Elements (ENCODE) data and formaldehyde-assisted isolation of regulatory elements sequencing analysis of OCPTs ( Supplementary Methods ). We observed no evidence of putative regulatory elements coinciding with rs12942666 or correlated SNPs ( Fig. 3a ). A map of regulatory elements in the entire 1-MB region can be seen in Supplementary Fig. 5c–f . We subsequently used in silico tools (ANNOVAR [23] , SNPinfo [24] and SNPnexus [25] ) to evaluate the putative function of possible causal SNPs ( Supplementary Methods ). Of 50 SNPs with possible functional roles, more than 30 reside in putative transcription factor binding sites (TFBS) within or near PLEKHM1 or ARHGAP27 ; 12 SNPs may affect methylation or miRNA binding, and two are non-synonymous coding variants predicted to be of no functional significance ( Supplementary Table S2 ). 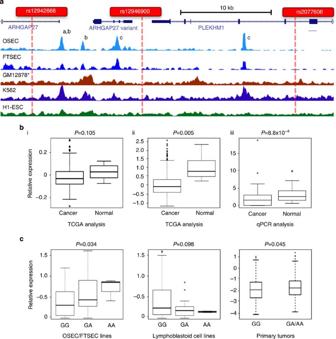Figure 3: The non-coding landscape and eQTL associations for the rs2077606 susceptibility SNP at 17q21.31. (a) Analysis of the chromatin landscape atARHGAP27andPLEKHM1in normal ovarian surface epithelial and fallopian tube secretory epithelial cells (OSECs/FTSECs) by formaldehyde-assisted isolation of regulatory elements sequencing (FAIRE-seq). Alignment with ENCODE FAIRE-seq tracks (shown) and ChIP-seq tracks (not shown) from non-EOC-related cell lines reveals open chromatin peaks corresponding to (a) promoters (b) CTCF insulator binding sites and (c) H3K4me3 signals, suggestive of a dynamic regulatory region. An H3K4me3 signal at a codingARHGAP27mRNA variant (c) located between the genes is highly pronounced in OSEC/FTSEC, suggesting tissue-specific expression and function. Several of the top-ranking SNPs fall within TFBS (Supplementary Table S2). rs12942666 did not coincide with TFBS, but tightly linked SNPs, rs12946900 and rs2077606 fell within predicted binding sites for SPIB and ZEB1, respectively. (b) We analysed the expression ofSPIBandZEB1in primary high-grade serous tumours from TCGA and found (i) no significant change inSPIBexpression but (ii) significant downregulation ofZEB1in tumours compared with normal tissues. (iii) QPCR analysis ofZEB1expression in 73 OCPT and 50 EOC cell lines supported the finding thatZEB1expression is lower in cancer cell lines compared with normal precursor tissues. (c) eQTL analysis in OSECs/FTSECs for different alleles of rs2077606. (i) There was a significant eQTL forARHGAP27, with the minor (A) allele being associated with increasedARHGAP27expression. (ii) There was no evidence of an association between rs2077606 genotypes andARHGAP27expression in lymphoblastoid cell lines, suggesting this association may be tissue-specific. (iii) We observed a borderline significant eQTL association betweenZEB1mRNA and rs2077606 in tumours from TCGA, with the minor risk allele also associated with lower expression. Figure 3: The non-coding landscape and eQTL associations for the rs2077606 susceptibility SNP at 17q21.31. ( a ) Analysis of the chromatin landscape at ARHGAP27 and PLEKHM1 in normal ovarian surface epithelial and fallopian tube secretory epithelial cells (OSECs/FTSECs) by formaldehyde-assisted isolation of regulatory elements sequencing (FAIRE-seq). Alignment with ENCODE FAIRE-seq tracks (shown) and ChIP-seq tracks (not shown) from non-EOC-related cell lines reveals open chromatin peaks corresponding to (a) promoters (b) CTCF insulator binding sites and (c) H3K4me3 signals, suggestive of a dynamic regulatory region. An H3K4me3 signal at a coding ARHGAP27 mRNA variant (c) located between the genes is highly pronounced in OSEC/FTSEC, suggesting tissue-specific expression and function. Several of the top-ranking SNPs fall within TFBS ( Supplementary Table S2 ). rs12942666 did not coincide with TFBS, but tightly linked SNPs, rs12946900 and rs2077606 fell within predicted binding sites for SPIB and ZEB1, respectively. ( b ) We analysed the expression of SPIB and ZEB1 in primary high-grade serous tumours from TCGA and found (i) no significant change in SPIB expression but (ii) significant downregulation of ZEB1 in tumours compared with normal tissues. (iii) QPCR analysis of ZEB1 expression in 73 OCPT and 50 EOC cell lines supported the finding that ZEB1 expression is lower in cancer cell lines compared with normal precursor tissues. ( c ) eQTL analysis in OSECs/FTSECs for different alleles of rs2077606. (i) There was a significant eQTL for ARHGAP27 , with the minor (A) allele being associated with increased ARHGAP27 expression. (ii) There was no evidence of an association between rs2077606 genotypes and ARHGAP27 expression in lymphoblastoid cell lines, suggesting this association may be tissue-specific. (iii) We observed a borderline significant eQTL association between ZEB1 mRNA and rs2077606 in tumours from TCGA, with the minor risk allele also associated with lower expression. Full size image As most of the top-ranked 17q21.31 SNPs with putative functions (including two of the top directly genotyped SNPs, rs2077606 and rs17631303) are predicted to lie in TFBS ( Supplementary Table S2 ), we used the in silico tool, JASPAR [26] , to further examine TFBS coinciding with these SNPs. Two SNPs scored high in this analysis ( Supplementary Table S5 ); the first, rs12946900, lies in a GAGGAA motif and canonical binding site for SPIB , an Ets family member [27] . Ets factors have been implicated in the development of ovarian cancer and other malignancies [28] , but little evidence supports a specific role for SPIB in EOC aetiology. The second hit was for rs2077606, which lies in an E-box motif CACCTG at the canonical binding site for ZEB1 (chr. 10p11.2), a zinc-finger E-box binding transcription factor that represses E-cadherin [29] , [30] and contributes to epithelial–mesenchymal transition in EOCs [31] . We analysed expression of SPIB and ZEB1 in primary ovarian cancers using TCGA data; we found no significant difference in SPIB expression in tumours compared with normal tissues ( Fig. 3bi ). In contrast, ZEB1 expression was significantly lower in primary HGS-EOCs compared with normal tissues ( P =0.005) ( Fig. 3bii ). We validated this finding using qPCR analysis in 123 EOC and OCPT cell lines ( P =8.8 × 10 − 4 ) ( Fig. 3biii ). As rs2077606 lies within an intron of PLEKHM1 , this gene is a candidate target for ZEB1 binding at this site. Our eQTL analysis also suggests ARHGAP27 is a strong candidate ZEB1 target at this locus; ARHGAP27 expression is highest in OCPT cell lines carrying the minor allele of rs2077606 ( P =0.034) ( Fig. 3ci ). Although we observed no eQTL associations between rs2077606 and ZEB1 expression in lymphoblastoid cell lines ( Fig. 3cii ), we found evidence of eQTL between rs2077606 and ZEB1 expression in HGS-EOCs ( P =0.045) ( Fig. 3ciii ). ZEB1 binding at the site of the common allele is predicted to repress gene expression whereas loss of ZEB1 binding conferred by the minor allele may enable expression of ARHGAP27 , consistent with the eQTL association in OCPTs ( Fig. 3ci ). Although these data support a repressor role for ZEB1 in EOC development and suggest ARHGAP27 may be a functional target of rs2077606 (or a correlated SNP) in OCPTs through trans-regulatory interactions with ZEB1, it is important to investigate additional hypotheses as we continue to narrow down the list of target susceptibility genes, SNPs, and regulatory mechanisms that contribute to EOC susceptibility at this locus. The present study represents the largest, most comprehensive investigation of the association between putative miRSNPs in the 3′UTR and cancer risk. This and the systematic follow-up to evaluate associations with EOC risk for non-miRSNPs in the region identified 17q21.31 as a new susceptibility locus for EOC. Although the miRSNPs identified here may have some biological significance, our findings suggest that other types of variants in non-coding DNA, especially non-miRSNPs at the 17q21.31 locus, are stronger contributors to EOC risk. It is possible, however, that highly significant miRSNPs exist that were not identified in our study because (a) they were not pre-selected for evaluation (that is, they do not reside in a binding site involving miRNAs or genes with known relevance to EOC, or they reside in regions other than the 3′UTR [3] , [4] ) and/or (b) they were very rare and could not be designed or detected with our genotyping platform and sample size, respectively. Despite these limitations, the homogeneity between studies of varying designs and populations in the OCAC and the genome-wide levels of statistical significance imply that all detected associations are robust. Furthermore, molecular correlative analyses of genes within the region suggest that cis -acting genetic variants influencing non-coding DNA regulatory elements, miRNAs and/or methylation underlie disease susceptibility at the 17q21.31 locus. Finally, these studies point to a subset of candidate genes (that is, PLEKHM1 , ARHGAP27 ) and a transcription factor (that is, ZEB1) that may influence EOC initiation and development. This novel locus is one of eleven loci now identified that contains common genetic variants conferring low penetrance susceptibility to EOC in the general population [17] , [32] , [33] , [34] . Genetic variants at several of these loci influence risks of more than one cancer type, suggesting that several cancers may share common mechanisms. For example, alleles at 5p15.33 and 19p13.1 are associated with estrogen-receptor-negative breast cancer and serous EOC susceptibility [32] , [35] , and variants at 8q24 are associated with risk of EOC and other cancers [17] , [36] . Genetic variation at 17q21.31 is also associated with frontotemporal dementia–spectrum disorders, Parkinson’s disease, developmental delay and alopecia [37] , [38] , [39] , [40] , [41] , [42] . Through COGS, the CIMBA also recently identified 17q21.31 variants that modify EOC risk in BRCA1 and BRCA2 carriers ( P <10 −8 in BRCA1/2 combined) [16] . In particular, rs17631303, which is perfectly correlated with rs2077606 and rs12942666, was among the top-ranking SNPs detected by CIMBA [16] . Consistent with our findings, CIMBA also provide data that suggest EOC risk is associated with altered expression of one or more genes in the 17q21.31 region [16] . Thus, results from this large-scale collaboration support a role for this locus in both BRCA1/2 - and non- BRCA1/2 -mediated EOC development. Before these findings can be integrated with variants from other confirmed loci and non-genetic factors to predict women at greatest risk of developing EOC and provide options for medical management of these risks, continued efforts will be needed to fine map the 17q21.31 region and to fully characterize the functional and mechanistic effects of potential causal SNPs in disease aetiology and development. Study population Forty-three individual OCAC studies contributed samples and data to the COGS initiative. Nine of the 43 participating studies were case-only (GRR, HSK, LAX, ORE, PVD, RMH, SOC, SRO, UKR); cases from these studies were pooled with case–control studies from the same geographic region. The two national Australian case–control studies were combined into a single study to create 34 case–control sets. Details regarding the 43 participating OCAC studies are summarized in Supplementary Table S1 . Briefly, cases were women diagnosed with histologically confirmed primary EOC (invasive or low malignant potential), fallopian tube cancer or primary peritoneal cancer ascertained from population- and hospital-based studies and cancer registries. The majority of OCAC cases (>90%) do not have a family history of ovarian or breast cancer in a first-degree relative, and most have not been tested for BRCA1/2 mutations as a part of their parent study. Controls were women without a current or prior history of ovarian cancer with at least one ovary intact at the reference date. All studies had data on disease status, age at diagnosis/interview, self-reported racial group and histologic subtype. Most studies frequency-matched cases and controls on age group and race. Selection of candidate genes and SNPs To increase the likelihood of identifying miRSNPs with biological relevance to EOC, we reviewed published literature and consulted public databases to generate two lists of candidate genes: (1) 55 miRNAs reported to be deregulated in EOC tumours compared with normal tissue in at least one study [43] , [44] , [45] , [46] , and (2) 665 genes implicated in the pathogenesis of EOC through gene expression analyses [47] , [48] , somatic mutations [49] , or genetic association studies [50] , [51] . Many genes were identified through the Gene Prospector database [51] , a web-based application that selects and prioritizes potential disease-related genes using a highly curated, up-to-date database of genetic association studies. Using each candidate gene list as input, we identified putative sites of miRNA:mRNA binding with the computational prediction algorithms TargetScan version 5.1 (refs 10 , 11 ) and PicTar [12] , [13] ( Supplementary Methods ). Each algorithm generated start and end coordinates for regions of miRNA binding, and database SNP [52] version 129 was mined to identify SNPs falling within the designated binding regions. Of 3,246 unique miRSNPs that were identified, 1,102 obtained adequate design scores using Illumina’s Assay Design Tool. The majority ( n =1,085, 98.5%) of the 1,102 SNPs resided in predicted sites of miRNA binding (and therefore represent miRSNPs), while the remainder ( n =17) are tagSNPs ( r 2 >0.80) for miRSNPs that were not designable or had poor-to-moderate design scores. Ninety-nine of the 1102 SNPs failed during custom assay development, leaving a total of 1,003 SNPs that were designed and genotyped. Genotyping and QC The candidate miRSNPs selected for the current investigation were genotyped using a custom Illumina Infinium iSelect Array as part of the international COGS, an effort to evaluate 211,155 genetic variants for association with the risk of ovarian, breast and prostate cancer. Samples and data were included from several consortia, including OCAC, the Breast Cancer Association Consortium, the Consortium of Investigators of Modifiers of BRCA1/2 (CIMBA) and the Prostate Cancer Association Group to Investigate Cancer-Associated Alterations in the Genome (PRACTICAL). Although one of the primary goals of COGS was to replicate and fine-map findings from pooled GWAS from each consortia, this effort also aimed to genotype candidate SNPs of interest (such as the miRSNPs). The genotyping and QC process has been described recently in our report of OCAC’s pooled GWAS findings [34] . Briefly, COGS genotyping was conducted at six centres, two of which were used for OCAC samples: McGill University and Génome Québec Innovation Centre (Montréal, Canada) ( n =19,806) and Mayo Clinic Medical Genomics Facility ( n =27,824). Each 96-well plate contained 250 ng genomic DNA (or 500 ng whole genome-amplified DNA). Raw intensity data files were sent to the COGS data coordination centre at the University of Cambridge for genotype calling and QC using the GenCall algorithm. Sample QC One thousand two hundred and seventy-three OCAC samples were genotyped in duplicate. Genotypes were discordant for greater than 40 per cent of SNPs for 22 pairs. For the remaining 1,251 pairs, concordance was greater than 99.6 per cent. In addition, we identified 245 pairs of samples that were unexpected genotypic duplicates. Of these, 137 were phenotypic duplicates and judged to be from the same individual. We used identity-by-state to identify 618 pairs of first-degree relatives. Samples were excluded according to the following criteria: (1) 1,133 samples with a conversion rate (the proportion of SNPs successfully called per sample) of less than 95 per cent; (2) 169 samples with heterozygosity >5 s.d’s from the intercontinental ancestry-specific mean heterozygosity; (3) 65 samples with ambiguous sex; (4) 269 samples with the lowest call rate from a first-degree relative pair; (5) 1,686 samples that were either duplicate samples that were non-concordant for genotype or genotypic duplicates that were not concordant for phenotype. A total of 44,308 eligible subjects including 18,174 cases and 26,134 controls were available for analysis. SNP QC The process of SNP selection by the participating consortia has been summarized previously [34] . In total, 211,155 SNP assays were successfully designed, including 23,239 SNPs nominated by OCAC. Overall, 94.5% of OCAC-nominated SNPs passed QC. SNPs were excluded if: (1) the call rate was <95% with MAF>5% or <99% with MAF<5% ( n =5,201); (2) they were monomorphic upon clustering ( n =2,587); (3) P -values of HWE in controls were <10 −7 ( n =2,914); (4) there was greater than 2% discordance in duplicate pairs ( n =22); (5) no genotypes were called ( n =1,311). Of 1,003 candidate miRSNPs genotyped, 767 passed QC criteria and were available for analysis; the majority of miRSNPs that were excluded were monomorphic ( n =158, 67%). Genotype intensity cluster plots were visually inspected for the most strongly associated SNPs. Population stratification HapMap DNA samples for European (CEU, n =60), African (YRI, n =53) and Asian (JPT+CHB, n= 88) populations were also genotyped using the COGS iSelect. We used the program LAMP [53] to estimate intercontinental ancestry based on the HapMap (release no. 23) genotype frequency data for these three populations. Eligible subjects with >90 per cent. European ancestry were defined as European ( n =39,773) and those with greater than 80 per cent. Asian or African ancestry were defined as Asian ( n =2,382) or African, respectively ( n =387). All other subjects were defined as being of mixed ancestry ( n =1,766). We then used a set of 37,000 unlinked markers to perform principal components analysis within each major population subgroup. To enable this analysis on very large sample sizes, we used an in-house program written in C++ using the Intel MKL libraries for eigenvectors (available at http://ccge.medschl.cam.ac.uk/software/ ). Tests of association We used unconditional logistic regression treating the number of minor alleles carried as an ordinal variable (log-additive model) to evaluate the association between each SNP and EOC risk. Separate analyses were carried out for each ancestry group. The model for European subjects was adjusted for population substructure by including the first five eigenvalues from the principal components analysis. African- and Asian ancestry-specific estimates were obtained after adjustment for the first two components representing each respective ancestry. Due to the heterogeneous nature of EOC, subgroup analysis was conducted to estimate genotype-specific ORs for serous carcinomas (the most predominant histologic subtype) and the three other main histological subtypes of EOC: endometrioid, mucinous and clear cell. Separate analyses were also carried out for each study site, and site-specific ORs were combined using a fixed-effect meta-analysis. The I 2 test of heterogeneity was estimated to quantify the proportion of total variation due to heterogeneity across studies, and the heterogeneity of ORs between studies was tested with Cochran’s Q statistic. The R statistical package ‘r-meta’ was used to generate forest plots. Statistical analysis was conducted in PLINK [54] . Imputation of genotypes at 17q21.31 To increase genomic coverage, we imputed genotype data for the 17q21.31 region (chr17: 40,099,001–44,900,000, human genome build 37) with IMPUTE2.2 (ref. 55 ) using phase 1 haplotype data from the January 2012 release of the 1,000 genome project data [15] . For each imputed genotype the expected number of minor alleles carried was estimated (as weights). IMPUTE provides estimated allele dosage for SNPs that were not genotyped and for samples with missing data for directly genotyped SNPs. Imputation accuracy was estimated using an r 2 quality metric. We excluded imputed SNPs from analysis where the estimated accuracy of imputation was low ( r 2 <0.3). Functional studies and in silico analysis of publicly available data sets We performed the following assays for each gene in the 1-MB region centred on the most significant SNP at the 17q21.31 locus (see Supplementary Methods ): gene expression analysis in EOC cell lines ( n =51) compared with normal cell lines from OCPTs [56] , including ovarian surface epithelial cells and fallopian tube secretory epithelial cells ( n =73) and CpG island methylation analysis in HGS ovarian cancer (HGS-EOC) tissues ( n =106) and normal tissues ( n =7). Genes in the region were also evaluated in silico by mining publicly available molecular data generated for primary EOCs and other cancer types, including TCGA analysis of 568 HGS EOCs [18] , the Gene Expression Omnibus series GSE18520 data set of 53 HGS EOCs [19] and the Catalogue Of Somatic Mutations in Cancer database [20] . We used these data to (1) compare gene expression between (a) EOC cell lines and normal cell lines and (b) tumour tissue and normal tissue from TCGA, (2) to compare gene methylation status in HGS-EOCs and normal tissue, (3) to conduct gene eQTL analyses to evaluate genotype–gene expression associations in normal OCPTs, lymphoblastoid cells and HGS-EOCs and (4) to conduct methylation quantitative trait locus analyses in HGS-EOCs to evaluate genotype–gene methylation associations. Data from ENCODE [57] were used to evaluate the overlap between regulatory elements in non-coding regions and risk-associated SNPs. ENCODE describes regulatory DNA elements (for example, enhancers, insulators and promotors) and non-coding RNAs (for example, miRNAs, long non-coding and piwi-interacting RNAs) that may be targets for susceptibility alleles. However, ENCODE does not include data for EOC-associated tissues, and activity of such regulatory elements often varies in a tissue-specific manner [57] , [58] . Therefore, we profiled the spectrum of non-coding regulatory elements in ovarian surface epithelial cells and fallopian tube secretory epithelial cells using a combination of formaldehyde-assisted isolation of regulatory elements sequencing and RNA sequencing ( Supplementary Methods ). How to cite this article: Permuth-Wey, J. et al . Identification and molecular characterization of a new ovarian cancer susceptibility locus at 17q21.31. Nat. Commun. 4:1627 doi: 10.1038/ncomms2613 (2013).